White matter in the older brain is more plastic than in the younger brain Visual perceptual learning (VPL) with younger subjects is associated with changes in functional activation of the early visual cortex. Although overall brain properties decline with age, it is unclear whether these declines are associated with visual perceptual learning. Here we use diffusion tensor imaging to test whether changes in white matter are involved in VPL for older adults. After training on a texture discrimination task for three daily sessions, both older and younger subjects show performance improvements. While the older subjects show significant changes in fractional anisotropy (FA) in the white matter beneath the early visual cortex after training, no significant change in FA is observed for younger subjects. These results suggest that the mechanism for VPL in older individuals is considerably different from that in younger individuals and that VPL of older individuals involves reorganization of white matter. Human brain processing declines with aging [1] , [2] , [3] . However, many age-related declines in function can be, to some degree, restored with practice. It is thought that such restoration is mainly due to reorganization of cortical areas [4] , [5] . Some visual tasks can be significantly improved by repeated practice. Such improvement is termed visual perceptual learning (VPL) [6] , [7] , [8] , [9] , [10] , [11] , [12] , [13] , [14] , [15] , [16] , [17] and is regarded as a manifestation of reorganization of visual and brain networks central to processing the task. It has been recently shown that VPL is also possible with older individuals (age 65+) [18] , [19] . This suggests that some visual functions that decline with age can be improved as a result of reorganization of networks in visual/brain processing. Given these improvements, an important question is what is the underlying neural mechanism of VPL with older adults? VPL with younger adults is strongly associated with changes in local networks in the early visual cortex [13] , [20] , [21] , [22] . Activation represented by blood oxygen level-dependent (BOLD) signals is changed in association with VPL [13] , [20] , [21] , [22] . Tuning properties of a trained feature based on action potentials of neurons in the localized region of V1 are changed [12] , [23] . These activation/activity changes, in association with learning, have been largely linked to synaptic efficacy changes [10] . However, because of age-related cortical changes, it is unclear whether changes in V1 occur in older adults as a result of VPL. First, cortical functions of older individuals may be too rigid to change due to reductions in grey matter volume [24] , [25] , [26] , [27] , [28] and thinning [27] , [29] , [30] , [31] . Second, a smaller magnitude of activation occurs for older as compared with younger adults when performing cognitive [32] and visual [33] tasks. Although it has been reported that age-related changes in occipital regions of both cortex/grey matter and white matter are smaller compared with other regions [34] , [35] , [36] , [37] , it has also been found that within the occipital region, aging reduces the surface size of earlier visual cortex to a greater degree than later visual cortical regions [38] . These findings raise the possibility that VPL for older adults may involve less plasticity in the early visual cortex, including synaptic changes as compared with younger adults. In addition to the cortical changes, changes in white matter have been found in association with learning. Previous research has found that skill acquisition and learning are associated with changes in fractional anisotropy (FA), which may reflect axonal diameter, myelin thickness, path geometry and fibre complexity in white matter [39] , [40] , [41] . This suggests that VPL, a type of skill learning, is achieved by enhanced efficiency in signal transmissions through axons [23] , which may be reflected by FA value changes as well as cortical plasticity including efficacy changes in synapses, which are reflected by changes in BOLD signals. These findings raise the possibility that, due to possible age-related declination or damage in the early visual cortex, the contribution of axonal processing in white matter to VPL significantly increases for older individuals. Given this possibility, it is predicted that the magnitude of FA changes in the occipital region should be significantly larger, for older as compared with younger adults, due to VPL training. In the current study, we conducted a brain imaging experiment with older and younger adults to test this possibility. As a result, we have found that the magnitude of FA changes in the occipital region due to VPL training is significantly larger for older than in younger adults. This finding suggests that underlying neural mechanisms associated with VPL training is changed by aging, and that VPL of older adults involves reorganization of white matter beneath the early visual cortex. Behavioural evidence for VPL in older adults Older subjects (see Methods for more details) participated in two magnetic resonance imaging (MRI) sessions, between which there were three behavioural training sessions that occurred within a 7-day period ( Fig. 1a ). During the behavioural training sessions, the subjects were trained with texture discrimination task (TDT; see Methods for more details), a task that is commonly used in VPL research [13] , [18] , [20] , [22] , [42] , [43] , [44] , [45] , and known to lead to VPL with a strong specificity in the trained visual location. On each trial, a texture display made of numerous line elements was presented ( Fig. 1b ). The subject’s main task was to report the orientation (vertical or horizontal) of the target, which consisted of five obliquely oriented lines, against the background, which consisted of horizontally oriented lines. The stimulus-to-mask onset asynchrony (SOA)—the time interval between the onset of the target display and the onset of masking pattern—was varied across blocks. The SOA that induced the 80% correct responses was defined as the threshold SOA, and was the primary behavioural measure. 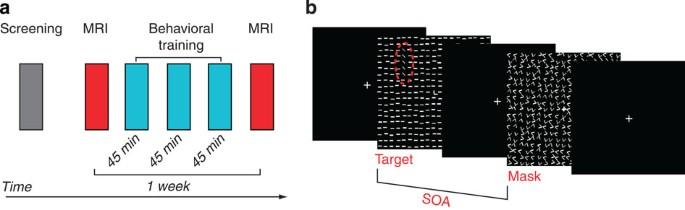Figure 1: Experimental procedure. (a) The complete experimental procedure. (b) The procedure of each trial. The time interval between the onsets of a target display and a mask (SOA) was varied. The red dotted ellipse indicates the target location, it is for an illustrative purpose and did not appear in the experiment. Figure 1: Experimental procedure. ( a ) The complete experimental procedure. ( b ) The procedure of each trial. The time interval between the onsets of a target display and a mask (SOA) was varied. The red dotted ellipse indicates the target location, it is for an illustrative purpose and did not appear in the experiment. Full size image The mean threshold SOAs significantly decreased over the 3-day training (one-way repeated measures analysis of variance (ANOVA), the significant training effect, F(2, 34)=4.135, P =0.0247; Fig. 2a ). Moreover, the present VPL for the older subjects showed the trained-location specificity ( Fig. 2b ). While the behavioural training was conducted only in one visual field quadrant, in the pre- and post-training MRI scans, TDT targets were presented not only in the trained but also in an untrained quadrant of the visual field (untrained quadrant) as a control. A repeated measures ANOVA with two factors being time (pre/post) and location (trained/untrained) showed significant main effects of time (F(1,17)=43.62, P <0.001), location (F(1,17)=21.583, P <0.001) and a significant interaction between these variables (F(1,17)=13.969, P =0.001). The results replicate previous research indicating that VPL occurs for older subjects with trained-location specificity in learning [18] . 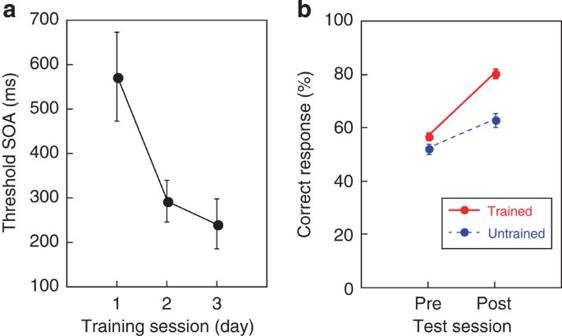Figure 2: Behavioural improvement in the older people. (a) The mean threshold SOA (±s.e.) as a function of training session (day) for the older group. (b) TDT performance during the two MRI sessions that showed the specificity in the training location (mean±s.e.).n=17 fora,b. Figure 2: Behavioural improvement in the older people. ( a ) The mean threshold SOA (±s.e.) as a function of training session (day) for the older group. ( b ) TDT performance during the two MRI sessions that showed the specificity in the training location (mean±s.e.). n =17 for a , b . Full size image White matter changes due to VPL in the older adults Previous research that investigated younger individuals has shown that cortical activation was significantly higher in the post-training scan, as compared with the pre-training scan in the region of V1 that retinotopically corresponds to the trained visual field quadrant (trained region in V1) [13] , [20] , [22] . Thus, we focused our investigation on the white matter underneath early visual cortex. To examine whether changes in the white matter occur in association with TDT, we measured the FA of the white matter volumes (volume of interest, VOI) beneath the trained and untrained regions in the early visual cortex that retinotopically correspond to the trained and untrained visual fields ( Fig. 3a–d ; for more details, see Methods). If FA changes are associated with VPL, then the changes should be larger in the white matter volume that is beneath the trained cortical region than for the volume beneath the untrained cortical region—a finding consistent with trained-location specificity for TDT. 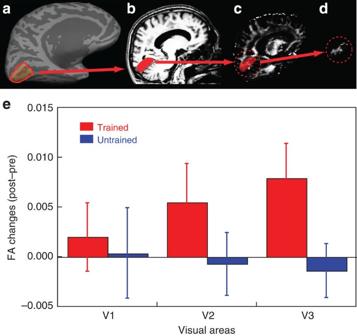Figure 3: FA changes in the older subjects. (a) An inflated format of the left brain of a subject and an ROI. First, using an inflated format of the brain61,62,70and a standard retinotopic mapping technique58, the visual borders of V1, V2 and V3 were determined to make cortical surface ROIs. The red line indicates one of the ROIs, the ventral cortical area, which retinotopically corresponds to a trained quadrant of visual field in V1. (b) Sagittal image of an anatomical MRI and the white matter VOI. The cortical ROI shown inawas converted into a folded format of the brain, and the white matter beneath the cortical ROI was selected as the white matter VOI (illustrated in red). (c) Raw FA map and white matter VOI. The rendered white matter VOI was applied to the raw FA map where FA value in each voxel is available. (d) Resultant FA volume within the white matter VOI. The FA values in voxels within the white matter VOI were averaged. Note the ROI and VOI oversimplified here for an illustrative purpose. (e) The mean subtraction (±s.e.,n=17) of FA obtained by DTI in the pre-training scan from that in the post-training scan for the trained region (red) and untrained region (blue) in V1, V2 and V3 for the older subjects. Figure 3: FA changes in the older subjects. ( a ) An inflated format of the left brain of a subject and an ROI. First, using an inflated format of the brain [61] , [62] , [70] and a standard retinotopic mapping technique [58] , the visual borders of V1, V2 and V3 were determined to make cortical surface ROIs. The red line indicates one of the ROIs, the ventral cortical area, which retinotopically corresponds to a trained quadrant of visual field in V1. ( b ) Sagittal image of an anatomical MRI and the white matter VOI. The cortical ROI shown in a was converted into a folded format of the brain, and the white matter beneath the cortical ROI was selected as the white matter VOI (illustrated in red). ( c ) Raw FA map and white matter VOI. The rendered white matter VOI was applied to the raw FA map where FA value in each voxel is available. ( d ) Resultant FA volume within the white matter VOI. The FA values in voxels within the white matter VOI were averaged. Note the ROI and VOI oversimplified here for an illustrative purpose. ( e ) The mean subtraction (±s.e., n =17) of FA obtained by DTI in the pre-training scan from that in the post-training scan for the trained region (red) and untrained region (blue) in V1, V2 and V3 for the older subjects. Full size image Figure 3e shows the mean FA changes from the pre- to post-training MRI scans within each of the white matter VOIs, which are beneath the cortical regions retinotopically corresponding to the trained and untrained visual field quadrants in V1, V2 and V3 in the older subjects. The FA of trained regions of V1, V2 and V3 was increased, whereas the FA of the untrained regions was not, in the post-training in comparison with the pre-training ( Fig. 3e ). Furthermore, the increase in FA change was largest in V3. We tested whether the FA values of the visual areas were significantly changed due to TDT training by three-way repeated measures ANOVA with factors being visual areas (V1/V2/V3), location (trained/untrained) and time (pre- and post-training). The results of ANOVA showed a significant main effect of visual areas (F(2,32)=8.448, P =0.0011), no significant main effects of location and the time factors, but a significant interaction between the location and the time (F(1,16)=6.455, P =0.0218). The significant main effect of visual areas and the significant interaction between the location and the time suggest that the FA values were increased in the white matter volume beneath the trained regions compared with the white matter volume beneath the untrained region, especially beneath the early visual areas of V3 due to the TDT training for older subjects. Small white matter changes due to VPL in younger adults Similar to the protocol for older adults, the younger subjects participated in two MRI sessions between which there were three behavioural training sessions that occurred over a 7-day period. As expected, the younger group showed learning during the training ( Fig. 4a ; one-way repeated measures ANOVA, a significant main effect of day, F(2,40)=28.360, P <0.001) and the learning was location specific ( Fig. 4b ), as indicated by comparing the pre- and post-training MRI sessions (two-way repeated measures ANOVA, a significant main effect of time (pre/post), F(1,20)=84.538, P <0.001, a significant main effect of location (trained/untrained), F(1,20)=38.505, P <0.001 and a significant interaction, F(1,20)=55.040, P <0.001). These results are in accord with previous work [13] , [20] , [22] . 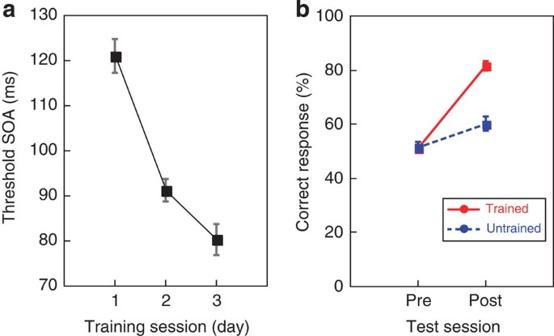Figure 4: Behavioural improvement in the younger people. (a) The mean threshold SOA (±s.e.) as a function of training session (day) for the younger group. (b) TDT performance during the two MRI sessions that showed the specificity in the training location (mean±s.e.).n=21 fora,b. Figure 4: Behavioural improvement in the younger people. ( a ) The mean threshold SOA (±s.e.) as a function of training session (day) for the younger group. ( b ) TDT performance during the two MRI sessions that showed the specificity in the training location (mean±s.e.). n =21 for a , b . Full size image Importantly, the FA changes in white matter volumes beneath the early visual cortex for younger subjects were much smaller than that for older subjects ( Fig. 5 ). While a smaller amount of changes in FA occurred for the younger group, significant BOLD signal increases took place in the trained regions of the early visual cortex with the younger group (see Supplementary Fig. 1 ). The BOLD signal results were consistent with previous studies [13] , [20] , [22] . 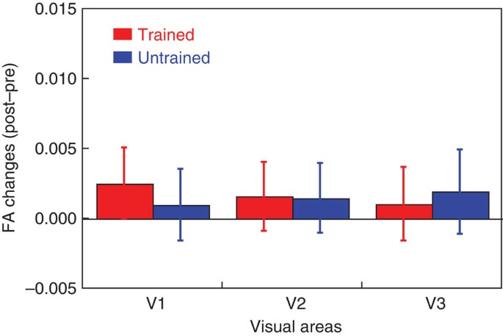Figure 5: FA changes in the younger subjects. The mean subtraction (±s.e.) of FA obtained by DTI in the pre-training scan from that in the post-training scan for the trained region (red) and untrained region (blue) in V1, V2 and V3 for the younger subjects (n=21). Figure 5: FA changes in the younger subjects. The mean subtraction (±s.e.) of FA obtained by DTI in the pre-training scan from that in the post-training scan for the trained region (red) and untrained region (blue) in V1, V2 and V3 for the younger subjects ( n =21). Full size image Comparison of groups Next we directly tested whether the degrees of FA changes due to perceptual learning were different between the age groups. We applied four-way repeated measures ANOVA with factors being age (older/younger), visual area (V1/V2/V3), location (trained/untrained) and time (pre/post). The results of the ANOVA showed a significant main effect of age (F(1,36)=14.810, P =0.0005), a significant main effect of visual area (F(2,72)=57.374, P <0.0001), a significant age × visual area interaction (F(2,72)=10.661, P =0.0001), a significant location × time interaction (F(1,36)=6.367, P =0.0162) and a significant age × location × time interaction (F(1,36)=5.245, P =0.028). These results suggest that the FA changes of the white matter volume beneath the early visual areas due to perceptual learning were (1) significantly larger for older as compared with younger subjects, (2) significantly larger in the trained location than in the untrained location and (3) significantly larger in the trained cortical region for older as compared with younger subjects. While the degree of FA changes was significantly different between the groups, the performance improvement was almost equivalent between the younger and older groups. Since different sets of SOAs were used between groups, we computed the performance improvement ratios for the two groups and compared them. The average performance improvement ratio for each group was obtained as a result of subtraction of the threshold SOA on day 3 from the threshold on day 1, divided by the threshold on day 1. The average performance improvement ratios were −28±8% (s.e.) for the older group and −30±4% (s.e.) for the younger group (see Supplementary Fig. 2 ). These ratios were not significantly different between the two groups (F(1,36)=0.119, NS). One may wonder whether the small FA changes with the younger group was due to other factors such as a ceiling effect and lower signal-to-noise ratio (SNR) of diffusion tensor imaging (DTI) data with younger adults. However, these factors are unlikely to account for the small FA changes with the younger group for the following two reasons. First, there seems to be no ceiling effect with FA distributions for either the younger or older group (see Supplementary Fig. 3 ). Second, the SNR (see Methods) of DTI data was actually better with younger adults than with older adults (see Supplementary Fig. 4 ). Correlation between V3 FA changes and performance improvement Results of our analyses showed that the FA values of white matter beneath V3 increased after the training with older subjects. The next question was whether the FA changes have any behavioural relevance. There are two types of behavioural measures: the threshold SOA during the 3-day training and the accuracy improvement between pre- and post-training MRI scans. Thus, we tested whether and, if so, how FA changes were related to each of the threshold SOA and accuracy changes. First, to investigate the relationship between the FA changes in V3 for older adults and the threshold SOA improvement during the 3-day training, we conducted binomial linear mixed-effect regression analyses with a maximal random effects structure [46] , [47] (see Supplementary Note 1 and Supplementary Tables 1–6 for more details). An initial model was fit that demonstrated that training improved performance ( P <0.05). A second model that included V3 FA change as a predictor of performance demonstrated that improved performance was associated with changes in V3 FA ( P <0.05) and that the effects of training depended on the amount of V3 FA change ( P <0.05). Moreover, after controlling for V3 FA change, the estimated magnitudes of the training effect were reduced. These results serve to demonstrate that V3 FA changes are a moderating, and potentially a partially mediating, factor for the effects of training. Second, we investigated whether the FA change beneath V3 is correlated with improved accuracy in the TDT (performance in the pre-MRI scan subtracted from that in the post-MRI scan) for older adults. A scatter plot between the improved accuracy and FA value showed a U-shaped curve tendency. A single linear regression did not fit very well ( r =−0.37, R 2 =0.1382, P =0.1416). Thus, we conducted a piecewise linear regression analysis in which the amount of improved accuracy that partitioned into two subgroups was determined to minimize the sum of squares of residuals of the linear regressions based on the two subgroups’ results for older subjects. The result was reasonably well fit to the data (coefficient of determination, R 2 =0.6196, P =0.0068; see Supplementary Fig. 5 ). These results indicate that there are two subgroups of subjects in older adults: good and poor learning groups. For the good learning group, the amount of accuracy improvement was positively correlated to the FA value change in V3, whereas for the poor learning group the amount of accuracy improvement was negatively correlated to the FA value change in V3. Other diffusivity parameters In addition to FA, we computed the mean diffusivity (MD), radial diffusivity (RD) and axial diffusivity (AXD) in each VOI for both younger and older groups (see Methods). However, none of MD, RD and AXD were significantly changed in association with perceptual learning in either the younger or older groups (see Supplementary Note 2 for more details). Next we tested whether FA changes were correlated with any of MD, RD and AXD in the older group. We found that only RD changes were modestly and negatively correlated with FA changes ( r =−0.54, P =0.027, uncorrected for multiple comparisons), indicating that older adults who tend to have increased FA after training tend to have decreased RD. Head motion Does a possible difference in head motions between the younger and older groups cause the differential results in FA values with the two groups? This is not likely for the following reasons. First, we calculated the FA values after motion correction procedures. Second, there was no significant difference in the overall sum of corrected head motions between the two groups (see Supplementary Note 3 for more details). Our results are unique and surprising. First, most previous evidence has shown that the brain of older adults tends to be less plastic than that of younger individuals [48] . However, results of the present study indicate that significant changes in FA in the white matter only occurred with older individuals. The results of the present study provide a strong case in which white matter beneath V3 is more readily changed with older as compared with younger individuals, although the lack of a significant white matter change with younger individuals due to VPL of TDT does not necessarily indicate that such changes never occur [49] . Second, the clear dissociation of the results for older and younger groups in terms of where the change takes place indicates that the mechanism for VPL is significantly different between the younger and older groups: While VPL in the younger brain is mainly associated with changes in activity/activation [13] , [20] , [22] , which we replicated in this study ( Supplementary Fig. 1 ), VPL in the older brain is mainly associated with changes in FA in the white matter ( Fig. 3e ). How can these results be interpreted? In the introduction, we raise the possibility that VPL of TDT can be achieved in two ways: one way is by improving axonal processing including myelination, axon caliber or crossing fibres in white matter [40] , [41] and the other way is by changing V1 cortical processing. The improvements in axonal processing may be reflected in FA changes in white matter, whereas the V1 changes may be reflected in BOLD signal changes [13] , [20] , [21] , [22] . The nature of TDT used in the present study may make older and younger adults use different weights on these two ways to improve TDT. TDT used in the present study requires segmentation of a target consisting of texture elements with one orientation from the background elements with a different orientation (see Fig. 1b ). One way to improve TDT performance is to better segment the target from the background. This could be accomplished by increasing the salience of the target while decreasing the salience of the background [43] . For younger adults, the requirement for differential processing of the target and background regions might be mainly accomplished by the strengthening of synaptic efficacies of excitatory processing for the target and inhibitory processing for the background, which may be reflected in greater BOLD activation in the trained region of V1 than in the untrained background region of V1 for younger individuals [13] , [20] , [22] ( Supplementary Fig. 1 ). On the other hand, for older adults, the differential requirements might be mainly reflected in the differential degrees of FA values that may reflect differences in axonal transmission related to myelination, axon caliber or crossing fibres in white matter [39] beneath the trained region and the untrained background region. In addition, results of our further analyses showed that FA increases tend to be correlated with RD decreases, suggesting that increases in myelination [50] , [51] , [52] , [53] may be associated with the FA increases. Why was the white matter change beneath V3 associated with VPL of TDT only for older and not for younger adults? There are several possible explanations. One explanation is due to the possible relative anti-aging resilience of the white matter beneath V3 as compared with V1. Results of the current experiment indicate that BOLD signal, which reflects neuronal activation, in the older individuals is not significantly greater in the trained region of V1 than the untrained region of V1, although significant difference in BOLD signals between these regions was found in the younger individuals [20] , [22] , [42] , [43] , [44] . In addition, no significant difference in FA changes was obtained between the trained and untrained regions in the white matter beneath V1/V2 in older subjects. These results suggest that both cortical processing of V1 and the axonal processing in the white matter beneath V1 declined by aging. If true, this could have made the contribution of axonal processing in the white matter beneath V3 to VPL greater than that of cortical processing and axonal processing beneath V1 for older individuals. The second explanation for the white matter change beneath V3 only for older adults is that the effect of VPL increases over the hierarchy of visual processing in both grey matter and white matter in older adults, and caused the larger FA changes beneath V3 than those beneath V1 and V2 in older adults as in Supplementary Fig. 7 . This raises the possibility that cortical regions higher in the hierarchy such as V4 or VO1 and the neighbouring white matter could show larger training effects. However, in the present study, we have not mapped higher visual areas, leaving this an open question. The third possibility is that the white matter in older adults is less optimal for such a demanding sensory task as TDT, as a result of normal aging. This may require white matter change to produce optimal learning. As a result, the effects of VPL by TDT may manifest more in white matter changes such as FA rather than BOLD signal changes with the older group. In contrast, the white matter of the younger adults may be nearly optimal for the task. Thus, changes due to VPL of TDT could occur in a grey matter region rather than a white matter region for younger individuals. These three possibilities are not contradictory to each other. However, the results of the present experiment cannot determine the validity of these possibilities. Thus, it is important that these hypotheses be tested in future research by conducting further systematic examinations of BOLD signal and FA values in the whole brain with younger and older individuals. As aforementioned, the result of the piecewise linear regression analysis ( Supplementary Fig. 5 ) indicates that the relationships between the amount of accuracy improvement of TDT and FA value changes are opposite between the old subjects whose accuracy improvement amount was higher than or equal to 22.8% (good learning group) and those whose accuracy improvement amount was lower than 22.8% (poor learning group). The good learning group tended to show a greater accuracy improvement with a larger FA value, whereas the poor learning group showed the opposite tendency. What are the underlying mechanisms to make good and poor learning groups out of older individuals? It is often the case that a greater FA value is correlated with performance increase from training [39] . The positive correlation between the amount of accuracy improvement and FA value with the good learning group in the current study may simply reflect improvements in axonal transmissions of neurons involved in target segmentation of TDT. On the other hand, there are multiple possible explanations for the negative correlation between the accuracy improvement and FA change with the poor learning group individuals. Previous studies have documented negative correlations between performance improvement and FA values [54] , [55] , [56] , [57] . Although clear underlying neural mechanisms are yet to be revealed, proposed possible factors include presence of crossing fibres [55] , [56] , [57] , increased axonal permeability [54] and increase in cell density or axonal/dendritic arborization [56] . It is possible that at least one of these factors acted against accuracy improvement in our study. However, the exact underlying biological mechanism for FA changes is still under investigation, thus leaving the interpretation of the increase or decrease in FA values unspecified. The present study indicates the importance of examining white matter changes in addition to grey mater cortical changes in the brain. While it has been indicated by many studies, including studies measuring BOLD signal, that the brain of older individuals is significantly less plastic, the results of the current study clearly show a higher degree of plasticity in the white matter of older individuals as compared with that of younger individuals. We suggest that such a higher degree of plasticity in white matter occurs to compensate for the smaller degree of plasticity shown in cortical processing. Subjects Eighteen older adults (11 females) aged 65–80 (mean=72.2, s.d.=5.4 years old) and 21 younger adults (7 females) aged 19–32 (mean=22.9, s.d.=2.9 years old) participated in this study. The sample size was determined based on a previous study [13] , [18] . DTI scan was not conducted with one of the older subjects due to a technical difficulty. Thus, a total number of 17 older subjects were used and DTI data were analysed. All subjects had normal or corrected-to-normal vision. Older subjects were recruited through the Harvard Cooperative on Aging, and were screened for dementia using the Mini Mental Status Examination. All subjects were healthy and were excluded if they had a dementia, a history of neurological and psychiatric disorder, or serious cardiovascular disease (see Supplementary Note 4 for more detailed screening results). All subjects gave written informed consent for their participation in the experimental protocol approved by the Institutional Review Board at Massachusetts General Hospital, University of California Riverside, Keio University and Boston University, where experiments were carried out. Experimental schedule Two MRI sessions including DTI were conducted ~1 week apart, and three training sessions were conducted between the two MRI sessions ( Fig. 1a ). Each MRI session lasted about 2 h, and each training session lasted about 45 min. All sessions were conducted on separate days, so that it took at least 5 days to complete the entire session. In addition, older subjects took the useful field of view test (UFOV, Visual Awareness Research Group Inc) after each MRI session to test whether attentional capacity changed as a result of TDT training [18] (see Supplementary Fig. 6 for the results). The UFOV results ruled out the possibility that the performance improvement with the older subjects was due to a change in attentional capacity, suggesting that the performance improvement in TDT involved the sensory level [18] , as has been found for younger individuals [13] , [20] , [22] . Texture discrimination task We employed the TDT [43] , in which a test stimulus was briefly presented and followed by a blank screen and a mask stimulus ( Fig. 1b ). The test stimulus consisted of a centrally located letter, either a ‘T’ or an ‘L’, and a peripherally positioned horizontal or vertical array of five diagonal bars on a background of horizontal bars. Each line segment was arranged within a 19-by-19 lattice in the area of an 18°-by-18°. Viewing distance was 57 cm in the training sessions as well as in the MRI sessions. Subjects answered whether the central letter was either T or L, and whether the target array was either horizontal or vertical by pressing buttons. The letter task was to ensure that subjects fixate at the centre of display. The orientation task was the main task, which improves with training. The target array was presented at 3–7° from the fixation in one of the visual quadrants. Task difficulty was determined by SOA. The task was easier with longer SOA. Throughout the training, a target was constantly presented within the same quadrant of the visual field, which was either in the left or right upper visual field. Assignment of the trained quadrant was counterbalanced across the subjects. A set of five SOAs was used in the training sessions. A set of (2,000, 1,000, 500, 250, 125 msec) or (500, 250, 200, 150, 125 msec) was used for older subjects. Which set to be used was predetermined by their performance in the screening session, in which 20 practice trials were conducted at the very beginning of the experiment. Subjects used the same SOA set during training. This arrangement was used to control for individual differences in task difficulty for older subjects. The SOA set was (200, 150, 100, 75, 50 msec) for younger subjects. The duration for the target stimulus was 100 msec for older subjects and 20 msec for younger subjects. Each training session consisted of 72 trials per SOA, resulting in a total of 360 trials per session. According to the original study [43] , the trials with the same SOA were blocked. The trials started with the longest SOA, which was gradually reduced in order. The 80% threshold SOA was estimated from a psychometric function where the percentage of correct responses was plotted against the various SOAs, according to the previous study [13] . Before and after the training, in the pre- and post-MRI scans, we also conducted TDT to test whether the learning was specific to the trained visual location. Target array was presented either in the upper left or in upper right visual quadrant; one of which was the trained quadrant as in the training session and the other was the control quadrant (untrained quadrant) that was not trained during the training session. Unlike the training session, only one SOA was used. The length of SOA was chosen from the initial screening session so that the correct response would be about 50–60% before the training for the older subjects. All younger subjects were tested with the SOA of 100 msec. The target durations were 100 msec for older subjects and 20 msec for younger subjects. There were a total of 96 trials for each of trained and untrained conditions. Functional MRI for retinotopic mapping We individually localized V1, V2 and V3 areas functionally using a standard flickering checkerboard pattern [13] , [42] , [58] to identify retinotopic representation of horizontal and vertical meridians of the visual fields, as well as the trained and untrained regions (3–7° eccentric from the fixation, in the upper left and the upper right visual field for either the trained and untrained regions, respectively). In the localizer scans, a total of five types of visual stimuli were presented with a grey background: (1) horizontal checkerboards (2 of 12° wedges centred on the horizontal meridian axis and symmetric to the fixation point at the centre of the display), (2) vertical checkerboards (2 of 24° wedges centred on the vertical meridian axis and symmetric to the fixation point), (3) checkerboards placed in trained and untrained visual fields, (4) a 168° wedge-shaped checkerboard placed in the upper visual field where the two parts that correspond to the trained and untrained regions were just in grey colour and (5) no checkerboard but a fixation. These stimuli were presented in counterbalanced orders in a blocked manner. Each block lasted 12 s. Each scan lasted 240 s, and was repeated twice. Retinotopic mapping was acquired using gradient echo EPI (Echo Planner Imaging) sequences (TR=2 s, TE=30 msec, flip angle=90°) for measurement of BOLD contrast. Thirty-three contiguous slices (3 × 3 × 3.5 mm 3 ) oriented parallel to the AC–PC plane were acquired to cover the entire brain. The slices were positioned using an automatic slice-positioning technique [59] . Data were analysed with the FS-FAST and FreeSurfer software ( http://surfer.nmr.mgh.harvard.edu/ ). All functional images were motion corrected [60] , spatially smoothed with a Gaussian kernel of 5.0 mm (full-width at half-maximum) and normalized individually across scans. MRI anatomical scan For an anatomical reconstruction [61] , [62] , three T1-weighted MR images (MPRAGE) were acquired (TR=2.531 s, TE=3.28 msec, flip angle=70, TI=1,100 msec, 256 slices, voxel size=1.3 × 1.3 × 1.0 mm 3 , resliced during analysis to 1 mm 3 ). DTI acquisition DTI data were acquired by using a single-shot echo-planar imaging sequence (60 directions [63] , uncorrected for slice angulation; b =700 s mm −2 , TR=7.98 s, TE=84 ms) [64] . The image matrix was 128 × 128 mm pixels, with a field of view of 256 × 256 mm (nominal resolution, 2.0 mm), with a partial Fourier factor of 6/8 phase applied. The bandwidth was 1,396 Hz per Px. Transverse sections of 2 mm thickness were acquired parallel to AC–PC plane with a total scan duration of 9 min 44 s. A total of 64 slices covered the entire cerebral cortex without gaps. One additional b =0 s mm −2 image was acquired for each slice. DTI data processing A diffusion-weighted data set was reconstructed [41] using FreeSurfer software. First, a motion/eddy current distortion correction procedure was conducted on diffusion volumes, using FLIRT [65] . Non-brain tissues were removed from the diffusion-weighted imaging using the Brain Extraction Tool (BET) from FSL [66] . General Linear Model (GLM) fit and tensor construction were conducted to extract diffusion parameters for later analyses. FA was calculated from the standard formula [67] . A apparent diffusion coefficient was defined as the mean of the three eigenvalues (or MD). The AXD was defined as the primary eigenvalue, and the RD was calculated as the average of the two smaller eigenvalues. The diffusion volumes were registered to the anatomical volume (see above) using a boundary-based registration procedure [68] . FA calculation for each VOI We determined the cortical region of interests (ROIs), beneath which the white matter VOIs were determined as follows (also see Fig. 3a–d ). First, cortical regions of 3–7° of eccentricity in V1, V2 and V3 were determined by functional localizer scans as described above. The ROIs were mapped onto the surface of an inflated brain [61] , [62] . Next, the cortical surface of each ROI was converted into a volume ROI, by filling into voxels up to 4 mm underneath the white matter/grey matter boundary to construct the white matter VOI. Because cortical surfaces were curved, some VOIs could be both underneath two regions such as V1 and V2, or V2 and V3. We identified such possible overlapping white matter volumes located between the borders (V1/V2 and V2/V3 volumes) and combined V1 and V1/V2 volumes as V1, and V2 and V2/V3 volumes as V2 so that no volumes belong to two different volumes. Raw FA map obtained from the DTI scans were co-registered to the subject’s anatomical volumes. So was the white matter VOI to calculate FAs within the white matter VOI. The FA values within the white matter VOI were averaged to represent the VOI, while only FA values larger than 0.2 were considered to correspond to white matter tissue, and included in the analysis. See Supplementary Figure 7A,B for the number of voxels above the 0.2 threshold, and Supplementary Fig. 7C,D for absolute FA values in VOIs for each group and time point. Other diffusivity calculations for VOIs MD, RD and AXD values were registered to the subject’s anatomical volumes [69] , and the values within the voxels whose FA values exceeded the threshold of 0.2 were averaged to represent the VOI. SNR calculations for VOIs SNR was computed using a low- b ( b =0 s mm −2 ) map. The low- b map was registered to the subject’s anatomical volumes. The low- b values within the voxels whose FA value exceeded the threshold of 0.2 were extracted. The mean and s.d. of the extracted low- b values were calculated for each VOI. The mean value divided by s.d. was determined as SNR. How to cite this article: Yotsumoto, Y. et al . White matter in the older brain is more plastic than in the younger brain. Nat. Commun. 5:5504 doi: 10.1038/ncomms6504 (2014).